Magnetic antibody-linked nanomatchmakers for therapeutic cell targeting Stem cell transplantation is a promising strategy for therapeutic cardiac regeneration, but current therapies are limited by inefficient interaction between potentially beneficial cells (either exogenously transplanted or endogenously recruited) and the injured tissue. Here we apply targeted nanomedicine to achieve in vivo cell-mediated tissue repair, imaging and localized enrichment without cellular transplantation. Iron nanoparticles are conjugated with two types of antibodies (one against antigens on therapeutic cells and the other directed at injured cells) to produce magnetic bifunctional cell engager (MagBICE). The antibodies link the therapeutic cells to the injured cells, whereas the iron core of MagBICE enables physical enrichment and imaging. We treat acute myocardial infarction by targeting exogenous bone marrow-derived stem cells (expressing CD45) or endogenous CD34-positive cells to injured cardiomyocytes (expressing myosin light chain. Targeting can be further enhanced by magnetic attraction, leading to augmented functional benefits. MagBICE represents a generalizable platform technology for regenerative medicine. Cell therapy has substantial promise in effecting regeneration [1] , [2] , [3] , [4] , [5] , [6] , but efficacy is limited by the need to deliver therapeutic cells in sufficient quantities to injured tissue [7] , [8] . Retention of cells delivered to the heart is generally <10% after several hours, regardless of the cell type and administration route. This may explain, at least in part, the small and inconsistent therapeutic benefit seen in clinical trials of bone marrow-derived stem cells for acute myocardial infarction (MI). Therefore, novel approaches are required to concentrate regenerative cells (either exogenous or endogenous) to their targets, and to engage them with the diseased tissue. Here we apply targeted nanomedicine to achieve in vivo cell-mediated tissue repair, imaging and localized enrichment without cellular transplantation. Iron nanoparticles are conjugated with two types of antibodies (one against antigens on therapeutic cells and the other directed at injured cells) to produce magnetic bifunctional cell engager (MagBICE). The antibodies link the therapeutic cells to the injured cells, whereas the iron core of MagBICE enables physical enrichment and imaging. We treated acute MI by targeting exogenous bone marrow-derived stem cells (expressing CD45) or endogenous CD34-positive cells to injured cardiomyocytes (expressing myosin light chain (MLC)). In vitro , MagBICE exhibits minimal cytotoxicity and specifically binds bone marrow-derived stem cells and injured cardiomyocytes, conjoining the two. In rats with MI, intravenously infused MagBICE concentrates in injured heart muscle, as visualized by magnetic resonance imaging (MRI). Furthermore, MagBICE captures circulating bone marrow-derived stem cells or endogenous CD34-positive cells and concentrates these cells in the injured heart tissue, reducing scar formation and improving pump function. Targeting can be further enhanced by magnetic attraction, leading to augmented functional benefits. Thus, we have achieved significant therapeutic efficacy, rivaling that of conventional cell therapy, with a novel intravenously infused nanoparticle. The magnetic nanomatchmaker concept is generalizable to a wide variety of disease targets. Synthesis of MagBICE and physicochemical properties The concept of MagBICE is illustrated schematically in Fig. 1a . Ferumoxytol (trade name: Feraheme (FH)) [9] is an iron nanoparticle coated with a carboxylated dextran polymer, enabling antibodies to be bound covalently by activating the carboxyl (COOH) groups with water-soluble carbodiimide 1-Ethyl-3-(3-Dimethylaminopropyl)carbodiimide (EDAC) reagent. The resultant active ester reacts with primary amines on the antibodies of interest. The first MagBICE particle tested here (MagBICE 1 ) was generated by conjugating anti-CD45 and anti-MLC antibodies to FH. Unconjugated FH and MagBICE 1 were visualized by cryo-transmission electron microscopy ( Fig. 1b ), with clear identification of the iron core and, for MagBICE 1 , the bound antibodies. The conjugation of both antibodies was further confirmed by immunofluorescent secondary antibodies targeting the primary antibodies on MagBICE 1 ( Fig. 1c ). The reduction of antibody concentration (measured by SDS PAGE and A280) in the post-conjugation solution confirms conjugation efficiency ( Fig. 1d,e ). Compared with FH, MagBICE 1 has a slightly larger size (mean±s.d. : 95.7±14.5 nm versus 25.2±5.0 nm; Fig. 1f and Supplementary Fig. 1 ) but a similar zeta potential (mean±s.d. : −9.6±1.5 mV versus −5.2±4.2 mV; Fig. 1g ). The addition of antibody linkers did not significantly change the slightly negative zeta-potential of FH, which is generally suitable for intravenous applications [10] , [11] . 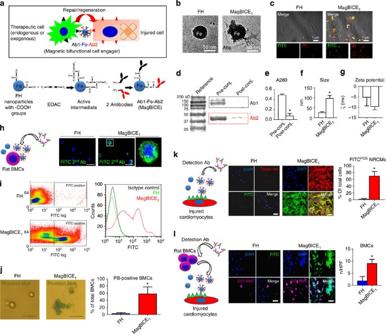Figure 1: Generation of MagBICE nanoparticles andin vitrobinding properties. (a) Schematic showing the concept of cell matchmaking by MagBICE and the preparation of MagBICE nanoparticles. (b) TEM images of unconjugated FH and MagBICE1nanoparticles. Conjugated antibodies (pointed as ‘Abs’) were negatively stained with uranyl acetate and iron oxide cores (indicated as ‘Fe’) in the complex were unstained. (c) Fluorescent micrographs showing clusters of unconjugated FH and MagBICE1stained with anti-mouse Texas-Red and anti-rabbit FITC secondary Abs, identifying the anti-MLC and anti-CD45 Abs on MagBICE1. (d) SDS–PAGE image showing the reduction of Ab amount in the supernatant after the conjugation reaction. (e) A280 protein concentrations in the pre- and post-conjugation solutions (P=0.0002;n=3). (f) Average hydrodynamic sizes of unconjugated FH and MagBICE1particles measured by a zeta metre (P=0.0013;n=3). (g) Average zeta potentials of unconjugated FH and MagBICE1particles measured by a zeta metre (P=0.1608;n=3). (h) Schematic showing the experiment where rat BMCs were incubated with FH or MagBICE1and then further incubated with secondary Abs (anti-rabbit FITC) for detection. Fluorescent microscopic images showing the binding of MagBICE1, but not FH, to rat BMCs (scale bars, 20 μm). (i) Flow cytometry analysis showing the specific binding of MagBICE1to rat BMCs. (j) Prussian blue staining of the iron cores showing the binding of MagBICE1, but not unconjugated FH, to rat BMCs (scale bars, 20 μm;P=0.0002;n=5). (k) Fluorescent microscopic images showing the binding of MagBICE1, but not unconjugated FH, to injured cardiomyocytes (NRCMs). The anti-MLC and anti-CD45 Abs on MagBICE1were detected by anti-mouse Texas-Red and anti-rabbit FITC secondary Abs, respectively (scale bars, 50 μm). The percentages of FITC-positive NRCMs were quantified (P<0.0001;n=5). (l) Fluorescent microscopic images showing MagBICE1conjoined rat BMCs (DiD-labelled; magenta) with injured NRCMs (green; scale bars, 50 μm). The numbers of BMCs attaching to NRCMs were quantified (P<0.0001;n=9). All data are mean±s.d. Comparisons between any two groups were performed using two-tailed unpaired Student’st-test. *P<0.05. DAPI, 4′,6-diamidino-2-phenylindole. Figure 1: Generation of MagBICE nanoparticles and in vitro binding properties. ( a ) Schematic showing the concept of cell matchmaking by MagBICE and the preparation of MagBICE nanoparticles. ( b ) TEM images of unconjugated FH and MagBICE 1 nanoparticles. Conjugated antibodies (pointed as ‘Abs’) were negatively stained with uranyl acetate and iron oxide cores (indicated as ‘Fe’) in the complex were unstained. ( c ) Fluorescent micrographs showing clusters of unconjugated FH and MagBICE 1 stained with anti-mouse Texas-Red and anti-rabbit FITC secondary Abs, identifying the anti-MLC and anti-CD45 Abs on MagBICE 1 . ( d ) SDS–PAGE image showing the reduction of Ab amount in the supernatant after the conjugation reaction. ( e ) A280 protein concentrations in the pre- and post-conjugation solutions ( P =0.0002; n =3). ( f ) Average hydrodynamic sizes of unconjugated FH and MagBICE 1 particles measured by a zeta metre ( P =0.0013; n =3). ( g ) Average zeta potentials of unconjugated FH and MagBICE 1 particles measured by a zeta metre ( P =0.1608; n =3). ( h ) Schematic showing the experiment where rat BMCs were incubated with FH or MagBICE 1 and then further incubated with secondary Abs (anti-rabbit FITC) for detection. Fluorescent microscopic images showing the binding of MagBICE 1 , but not FH, to rat BMCs (scale bars, 20 μm). ( i ) Flow cytometry analysis showing the specific binding of MagBICE 1 to rat BMCs. ( j ) Prussian blue staining of the iron cores showing the binding of MagBICE 1 , but not unconjugated FH, to rat BMCs (scale bars, 20 μm; P =0.0002; n =5). ( k ) Fluorescent microscopic images showing the binding of MagBICE 1 , but not unconjugated FH, to injured cardiomyocytes (NRCMs). The anti-MLC and anti-CD45 Abs on MagBICE 1 were detected by anti-mouse Texas-Red and anti-rabbit FITC secondary Abs, respectively (scale bars, 50 μm). The percentages of FITC-positive NRCMs were quantified ( P <0.0001; n =5). ( l ) Fluorescent microscopic images showing MagBICE 1 conjoined rat BMCs (DiD-labelled; magenta) with injured NRCMs (green; scale bars, 50 μm). The numbers of BMCs attaching to NRCMs were quantified ( P <0.0001; n =9). All data are mean±s.d. Comparisons between any two groups were performed using two-tailed unpaired Student’s t -test. * P <0.05. DAPI, 4′,6-diamidino-2-phenylindole. Full size image Binding and engaging activities in vitro The ability of MagBICE 1 to bind specifically to stem cells and injured heart muscle cells, and conjoin the two, was investigated in vitro using rat bone marrow mononuclear cells (BMCs) and neonatal rat cardiomyocytes (NRCMs). Confocal imaging ( Fig. 1h ), flow cytometry ( Fig. 1i ) and Prussian blue iron staining ( Fig. 1j ) confirmed that MagBICE 1 bound efficiently to rat BMCs, whereas unconjugated FH did not. An antibody stripping protocol ruled out any significant endocytosis of MagBICE 1 by BMCs ( Supplementary Fig. 2 ). NRCMs were lightly permeabilized to mimic membrane disruption secondary to ischemic injury; this maneuver exposes MLC, which is normally confined to the intracellular compartment. MagBICE 1 bound to injured NRCMs, whereas unconjugated FH did not (mean±s.d. : 69.5±14.0% versus 1.5±2.3% fluorescein isothiocyanate (FITC)-positive NRCMs, Fig. 1k ). Binding was specific to injured cells, as MagBICE 1 did not bind to healthy NRCMs ( Supplementary Fig. 3a ). To demonstrate conjoining, rat BMCs were co-cultured with injured NRCMs, in the presence of MagBICE 1 or FH. MagBICE 1 , but not FH, increased the number of BMCs attaching to injured cardiomyocytes (mean±s.d. : 9.0±1.7 versus 1.8±1.9 DiD-labelled BMCs per high power field (HPF), Fig. 1l ). A scrambled control of MagBICE null (FH conjugated with rabbit and mouse IgG isotype control antibodies) neither bound to injured NRCMs nor engaged them with BMCs, indicating that the binding/engaging effects of MagBICE 1 are specific ( Supplementary Fig. 3b ). The presence of MagBICE 1 did not affect NRCM viability (mean±s.d. : 6.8±3.2% versus 7.0±2.5% EthD-positive dead cells, Supplementary Fig. 4 ), BMC proliferation ( Supplementary Fig. 5 ) or BMC migration ( Supplementary Fig. 6 ), indicative of minimal cytotoxicity. Binding and engaging activities in vivo To test the injury-targeting and cell-engaging abilities of MagBICE 1 in vivo , MI was created by ischemia/reperfusion injury in rats ( Fig. 2a ). Cardiac MRI revealed that intravenously-delivered MagBICE 1 efficiently targeted to the injured myocardium, creating a signal void in T2* weighted MRI images (yellow arrows, Fig. 2b ). Unconjugated FH created a ‘hypointensity’ much smaller than MagBICE but slightly greater than that in the control group. Immunohistochemistry further confirmed the binding of MagBICE 1 , but not FH, to the infarct zone ( Fig. 2c ). Here we utilized a goat-FITC-conjugated anti-rabbit secondary antibody to detect the rabbit anti-CD45 antibody on MagBICE 1 . Specific FITC fluorescence was evident in the infarct zone of the MagBICE 1 -treated animals. High magnification revealed the globular morphology of MagBICE 1 (as detected by fluorophore-conjugated secondary antibody (green, Fig. 2c )) and its presence on the surface of cardiomyocytes (red, Fig. 2c ). The iron core of MagBICE 1 was visualized by Prussian blue staining ( Supplementary Fig. 7 ). Binding specificity was confirmed by the absence of MagBICE 1 in non-infarcted (remote) myocardium. MagBICE 1 infusion resulted in an increase of CD45-positive cells in the infarct area (mean±s.d. : 11.7±3.6 versus 1.9±1.9 cells per HPF, Fig. 2d ). MagBICE 1 did not exacerbate inflammation in the post-MI heart: the numbers of CD68-positive macrophages (magenta, Fig. 2e ) were similar in the three experimental groups. The majority of MagBICE 1 (green, Fig. 2e ) was bound to cardiomyocytes, although some had been internalized by macrophages as indicated by FITC (MagBICE 1 )/CD68 double-positive cells. In vitro , internalization of MagBICE 1 by isolated rat macrophages was minimal, as compared with larger iron beads (positive control) designed for endocytosis ( Supplementary Fig. 8 ). There was no sign of iron overload: infusion of MagBICE 1 did not elevate serum transferrin or ferritin levels ( Supplementary Figs 9 and 10 ), nor was there excessive free iron in the liver ( Supplementary Fig. 11 ). 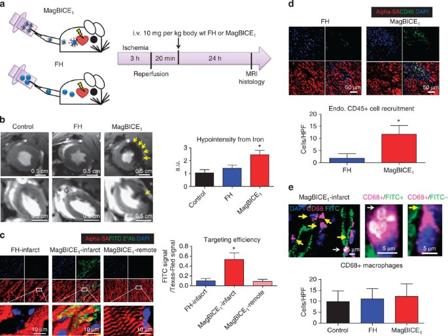Figure 2: MagBICE1targets injured myocardium and recruits endogenous cellsin vivo. (a) Schematic ofin vivotargeting experiment in rats with ischemia/injury injury. (b) T2* weighted MRI images showing the specific targeting of MagBICE1to injured myocardium. The presence of iron-created signal void (dark area; pointed with yellow arrows). The images were inverted so the signal void (dark area) from the iron signal led to higher value of ‘hypointensity’. The iron signal intensity of the heart anterior wall was quantified and normalized to adjacent tissue (P=0.0015;n=3 animals). *P<0.05 when compared with control. (c) Confocal microscopic images showing the co-localization of MagBICE1(green) with cardiomyocytes (red) in the infarct area. The binding of MagBICE1to healthy myocytes in the non-infarcted (remote) area was negligible (P<0.0001;n=3 animals and 6 microscopic fields). *P<0.05 when compared with FH-infarct. (d) Confocal microscopic images showing MagBICE1recruited endogenous CD45-positive cells (green) to the infarct area (P<0.0001;n=3 animals and 27 microscopic fields). *P<0.05. (e) Confocal microscopic images showing CD68-positive macrophages (magenta) in the infarct area. MagBICE1was detected by anti-rabbit FITC secondary antibodies (green). Most macrophages were MagBICE1-free (yellow arrows) but a few macrophages had endocytosized MagBICE1(white arrow). MagBICE1infusion did not increase the number of macrophages in the post-MI heart (P=0.5596;n=3 animals and 27 microscopic fields). All data are mean±s.d. Comparisons between any two groups were performed using two-tailed unpaired Student’st-test. Comparisons among more than two groups were performed using one-way ANOVA followed bypost-hocBonferroni test. DAPI, 4′,6-diamidino-2-phenylindole. Figure 2: MagBICE 1 targets injured myocardium and recruits endogenous cells in vivo . ( a ) Schematic of in vivo targeting experiment in rats with ischemia/injury injury. ( b ) T 2 * weighted MRI images showing the specific targeting of MagBICE 1 to injured myocardium. The presence of iron-created signal void (dark area; pointed with yellow arrows). The images were inverted so the signal void (dark area) from the iron signal led to higher value of ‘hypointensity’. The iron signal intensity of the heart anterior wall was quantified and normalized to adjacent tissue ( P =0.0015; n =3 animals). * P <0.05 when compared with control. ( c ) Confocal microscopic images showing the co-localization of MagBICE 1 (green) with cardiomyocytes (red) in the infarct area. The binding of MagBICE 1 to healthy myocytes in the non-infarcted (remote) area was negligible ( P <0.0001; n =3 animals and 6 microscopic fields). * P <0.05 when compared with FH-infarct. ( d ) Confocal microscopic images showing MagBICE 1 recruited endogenous CD45-positive cells (green) to the infarct area ( P <0.0001; n =3 animals and 27 microscopic fields). * P <0.05. ( e ) Confocal microscopic images showing CD68-positive macrophages (magenta) in the infarct area. MagBICE 1 was detected by anti-rabbit FITC secondary antibodies (green). Most macrophages were MagBICE 1 -free (yellow arrows) but a few macrophages had endocytosized MagBICE 1 (white arrow). MagBICE 1 infusion did not increase the number of macrophages in the post-MI heart ( P =0.5596; n =3 animals and 27 microscopic fields). All data are mean±s.d. Comparisons between any two groups were performed using two-tailed unpaired Student’s t -test. Comparisons among more than two groups were performed using one-way ANOVA followed by post-hoc Bonferroni test. DAPI, 4′,6-diamidino-2-phenylindole. Full size image Functional benefits of MagBICE 1 for BMC therapy Is MagBICE infusion capable of therapeutic cell targeting and regeneration of the injured tissue? To address this question, MagBICE 1 or FH was infused intravenously in rats with acute MI ( Fig. 3a,b ). Twenty minutes later, 2 million syngeneic DiI-labelled BMCs were infused to create circulating labelled stem cells. MagBICE 1 increased BMC targeting (red DiI signal) to the heart while decreasing off-target fluorescence in the lungs ( Fig. 3c ), as confirmed by histology showing that MagBICE 1 boosted the number of BMCs in the infarct zone (mean±s.d. : 33.1±14.7 versus 3.7±1.7 cells per HPF, Fig. 3d ). BMCs (red) coated with MagBICE 1 were generally co-localized with injured cardiomyocytes (green) in the infarct zone. Although fluorescent molecules leftover from dead BMCs may be taken up by the surrounding cells, the DiI fluorescence should still represent the amount of BMCs that were originally recruited (either dead or alive at 24 h). The engineered stem cell targeting and cell–cell coupling produced by MagBICE 1 led to therapeutic benefit. Masson's trichrome staining distinguishes viable tissue (red) from scar (blue, Fig. 3e ). Compared with the control group, scar mass was reduced (mean±s.d. : 23.6±7.2 versus 43.9±6.2 mg), as was scar size (mean±s.d. : 16.3±4.9% versus 35.1±10.4%; expressed as a percentage of the total left ventricular (LV) mass). Meanwhile, infarct wall thickness was greater (that is, better preserved) with MagBICE 1 +BMC infusion (mean±s.d. : 0.85±0.22 mm versus 0.41± 0.13 mm). Global pump function, as gauged by LV ejection fraction (LVEF), was indistinguishable among all three groups at baseline (24 h after MI), indicating similar degrees of injury ( Fig. 3f ; left, white bars). Four weeks later, LVEF was higher in MagBICE 1 +BMC infused animals than in those that had received saline infusion (mean±s.d. : 41.6±6.7% versus 26.7±2.8%, Fig. 3f ; left, black bars). Indeed, saline infusion had a negative treatment effect with decreasing LVEFs over time, whereas MagBICE 1 +BMC robustly preserved heart function (right, Fig. 3f ). Unconjugated FH+BMC infusion was not different from saline infusion in any measures, indicating that cell targeting to the injury zone is essential to therapeutic benefits. Histology revealed that MagBICE 1 +BMC infusion promoted angiogenesis as compared with the control group (mean±s.d. : 47.0±11.4 versus 15.3±4.7, Fig. 3g ), a well-known mechanism of benefit in BMC-based therapies [12] . Furthermore, more cardiomyocytes were present in the peri-infarct area of MagBICE 1 -treated hearts, consistent with de novo cardiomyogenesis and/or better preservation of cardiomyocytes at-risk after acute MI ( Supplementary Fig. 12 ). 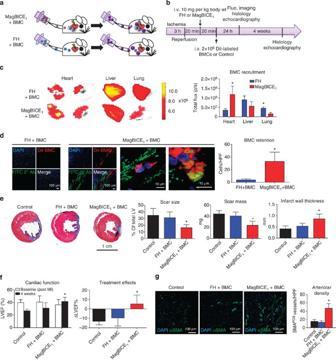Figure 3: MagBICE1infusion leads to therapeutic cell targeting and regeneration of injured heart tissue. (a,b) Schematic showing therapeutic efficacy studies of MagBICE1in rats with ischemia/injury injury. (c)Ex vivofluorescent imaging showing MagBICE1-targeted intravenously infused BMCs (DiI-labelled; red) to the heart (P=0.0344;n=3 animals) and decreased off-target retention in the lungs (P=0.0071;n=3 animals). *P<0.05 when compared with FH. (d) Confocal microscopic images confirming MagBICE1-enhanced BMC binding to the heart (P<0.0001;n=3 animals and nine microscopic fields). MagBICE1conjoined infused BMCs (red) with cardiomyocytes (green) in the infarct area. *P<0.05. (e) Masson’s trichrome images showing scar (blue) and viable (red) tissues in the heart 4 weeks post MI. MagBICE1+BMC therapy induced healing: scar size (P=0.0087;n=5 animals) and scar mass (P=0.0011;n=5 animals) were decreased, and infarct wall thickness was increased (P=0.0033; n=5 animals). *P<0.05 when compared with control. (f) Echocardiography showing no difference in LVEFs among the groups at baseline (P=0.6177;n=6 animals). Four weeks later, animals treated with MagBICE1+BMC had greater LVEFs than those received control or FH+BMC therapies (P=0.0037;n=6 animals), and greater treatment effects (change in LVEF over the 4-week time course;P=0.0019;n=6 animals). *P<0.05 when compared with control. (g) Confocal microscopic images showing MagBICE1+BMC therapy boosted angiogenesis in the post-MI heart (P<0.0001;n=3 animals and 27 microscopic fields). *P<0.05 when compared with control. All data are mean±s.d. Comparisons between any two groups were performed using two-tailed unpaired Student’st-test. Comparisons among more than two groups were performed using one-way ANOVA followed bypost-hocBonferroni test. DAPI, 4′,6-diamidino-2-phenylindole. Figure 3: MagBICE 1 infusion leads to therapeutic cell targeting and regeneration of injured heart tissue. ( a , b ) Schematic showing therapeutic efficacy studies of MagBICE 1 in rats with ischemia/injury injury. ( c ) Ex vivo fluorescent imaging showing MagBICE 1 -targeted intravenously infused BMCs (DiI-labelled; red) to the heart ( P =0.0344; n =3 animals) and decreased off-target retention in the lungs ( P =0.0071; n =3 animals). * P <0.05 when compared with FH. ( d ) Confocal microscopic images confirming MagBICE 1 -enhanced BMC binding to the heart ( P <0.0001; n =3 animals and nine microscopic fields). MagBICE 1 conjoined infused BMCs (red) with cardiomyocytes (green) in the infarct area. * P <0.05. ( e ) Masson’s trichrome images showing scar (blue) and viable (red) tissues in the heart 4 weeks post MI. MagBICE 1 +BMC therapy induced healing: scar size ( P =0.0087; n =5 animals) and scar mass ( P =0.0011; n =5 animals) were decreased, and infarct wall thickness was increased ( P =0.0033; n=5 animals). * P <0.05 when compared with control. ( f ) Echocardiography showing no difference in LVEFs among the groups at baseline ( P =0.6177; n =6 animals). Four weeks later, animals treated with MagBICE 1 +BMC had greater LVEFs than those received control or FH+BMC therapies ( P =0.0037; n =6 animals), and greater treatment effects (change in LVEF over the 4-week time course; P =0.0019; n =6 animals). * P <0.05 when compared with control. ( g ) Confocal microscopic images showing MagBICE 1 +BMC therapy boosted angiogenesis in the post-MI heart ( P <0.0001; n =3 animals and 27 microscopic fields). * P <0.05 when compared with control. All data are mean±s.d. Comparisons between any two groups were performed using two-tailed unpaired Student’s t -test. Comparisons among more than two groups were performed using one-way ANOVA followed by post-hoc Bonferroni test. DAPI, 4′,6-diamidino-2-phenylindole. Full size image Functional benefits of MagBICE 2 with magnetic targeting We next sought to address two new questions: (i) Is MagBICE capable of enriching endogenous stem cells in the infarct area and exerting therapeutic benefits similar to those of cell transplantation? (ii) Is the iron core of MagBICE potentially useful not only for imaging but also for physical enrichment by applying an external magnet [13] ? To address these questions, we created another MagBICE (MagBICE 2 ) by conjugating anti-CD34 and anti-MLC antibodies to FH. MagBICE 2 specifically binds to injured cardiomyocytes in vitro ( Supplementary Fig. 13 ). When delivered intravenously to rats post MI ( Fig. 4a ), MagBICE 2 homed to injured myocardium as evidenced by the localized MRI signal void ( Fig. 4b , MagBICE 2 ). Targeting was further enhanced by local application of a magnetic field ( Fig. 4b , MagBICE 2 +M). Peripheral blood mononuclear cells (PBMCs) were isolated 24 h after delivery of MagBICE 2 ; some PBMCs bound to the nanoparticles, with further enrichment by magnetically activated cell sorting ( Supplementary Fig. 14 ). Flow cytometry revealed these cells to be predominantly CD34 positive. Four weeks after treatment with MagBICE 2 , endogenous CD34 cells were enriched in the heart (7.8±2.6 cells per HPF versus 3.6±1.8 in saline controls or 3.1±1.6 with FH infusion). Such binding was further boosted by magnetic targeting (to 15.4±5.1 cells per HPF, Fig. 4c ). Administration of MagBICE 2 with magnetic targeting resulted in the greatest preservation of viable tissue in the risk region ( Fig. 4d ) and the highest cardiac function (LVEF; Fig. 4e ) at 4 weeks. Although treatment with MagBICE 2 improves outcomes even without magnetic targeting, focused physical attraction clearly enhances efficacy. 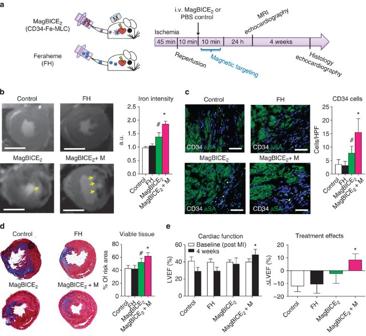Figure 4: MagBICE1infusion and magnetic targeting enrich endogenous stem cells in the infarct and ameliorate ventricular dysfunction. (a) Schematic showing therapeutic efficacy studies of MagBICE2(CD34-Fe-MLC) and magnetic targeting in rats with ischemia/reperfusion injury. (b) T2* weighted MRI images showing the specific targeting of MagBICE2to injured myocardium. The presence of iron-created signal void (dark area; pointed with yellow arrows). The iron signal intensity of the heart anterior wall was quantified and normalized to adjacent tissue (P<0.0001;n=3 animals). Scale bars, 0.5 cm. (c) Confocal microscopic images showing MagBICE2-recruited endogenous CD34-positive cells (white) to the infarct area (P<0.0036;n=3 animals and 27 microscopic fields). (d) Masson’s trichrome images showing scar (blue) and viable (red) tissues in the heart 4 weeks post MI. Infusion of MagBICE2with magnetic targeting preserved viable tissue in the risk region (P<0.0001;n=3 animals and nine sections). (e) Echocardiography reveals no difference in LVEFs among the groups at baseline (P=0.9424;n=6 animals). Four weeks later, animals treated with MagBICE2+Magnet had greater LVEFs than those received control or FH therapies (P<0.0001;n=6 animals), and greater treatment effects (change in LVEF over the 4-week time course;P<0.0001;n=6 animals).#P<0.05 when compared with control or FH group. *P<0.05 when compared with any other groups. Figure 4: MagBICE 1 infusion and magnetic targeting enrich endogenous stem cells in the infarct and ameliorate ventricular dysfunction. ( a ) Schematic showing therapeutic efficacy studies of MagBICE 2 (CD34-Fe-MLC) and magnetic targeting in rats with ischemia/reperfusion injury. ( b ) T 2 * weighted MRI images showing the specific targeting of MagBICE 2 to injured myocardium. The presence of iron-created signal void (dark area; pointed with yellow arrows). The iron signal intensity of the heart anterior wall was quantified and normalized to adjacent tissue ( P <0.0001; n =3 animals). Scale bars, 0.5 cm. ( c ) Confocal microscopic images showing MagBICE 2 -recruited endogenous CD34-positive cells (white) to the infarct area ( P <0.0036; n =3 animals and 27 microscopic fields). ( d ) Masson’s trichrome images showing scar (blue) and viable (red) tissues in the heart 4 weeks post MI. Infusion of MagBICE 2 with magnetic targeting preserved viable tissue in the risk region ( P <0.0001; n =3 animals and nine sections). ( e ) Echocardiography reveals no difference in LVEFs among the groups at baseline ( P =0.9424; n =6 animals). Four weeks later, animals treated with MagBICE 2 +Magnet had greater LVEFs than those received control or FH therapies ( P <0.0001; n =6 animals), and greater treatment effects (change in LVEF over the 4-week time course; P <0.0001; n =6 animals). # P <0.05 when compared with control or FH group. * P <0.05 when compared with any other groups. Full size image Currently, there are >30 Food and Drug Administration-approved antibody therapies [14] , including 10 blockbuster drugs. Most are for cancer therapy, for example, antibodies designed to recruit cytotoxic T cells to cancer cells. The latter principle utilizes the simpler entity of bispecific T-cell engager [15] , which consists of fused monoclonal antibody fragments without a magnetic core. MagBICE and bispecific T-cell engager are similar in that both exploit conjoined antibodies to achieve molecular co-localization. Bispecific proteins and antibodies have also been used to enhance stem cell targeting and tissue regeneration [16] , [17] , [18] , [19] . MagBICE, however, differs fundamentally from bispecific antibodies in that the iron core enables visualization of tissue localization by MRI and enhancement of targeting efficacy by local magnetic fields. These features may overcome some of the limitations of conventional cell therapy, including uncertainties in biodistribution and poor cell retention, even with local delivery [20] . Systemic delivery by intravenous infusion is minimally invasive, but suffers from paltry homing to the target organ [21] . Two prototypes of MagBICE target systematically delivered stem cells or endogenous stem cells to injured heart tissue, generating sizable therapeutic outcomes not dissimilar to those seen in preclinical models of direct BMC transplantation [22] , [23] . Compared with a previous report using bispecific antibody-armed BMCs [24] , our technology represents a qualitative step forward. First, the manipulating agent needs not be pre-armed with BMCs in vitro ; instead, MagBICE can capture endogenous BMCs in vivo , as we have shown with MagBICE 2. Moreover, the iron nanocore enables detection by MRI and physical (magnetic) enrichment. Our study also has several limitations. First, the hypoenhancement created by iron may distort the quality of MR images during the initial period after infusion. The degradation and absorption of iron should mitigate this problem over time. Second, MagBICE 2 alone produces only marginal functional benefit, further emphasizing the utility of synergistic magnetic targeting. It is possible that insufficient CD34 + cells are available in the circulation for MagBICE to capture, limiting therapeutic efficacy. We have not yet tested whether adjunctive bone marrow-stimulating agents such as granulocyte–colony-stimulating factor might enhance MagBICE efficacy, but such a conjecture merits future investigation. Third, in our study, MagBICE was delivered immediately after reperfusion in rats. In many clinical scenarios, a later time point of administration may be more realistic, but we have not yet studied the effects of delayed administration. Finally, we did not include a MagBICE null group in our animal studies. The nonspecific binding effects of MagBICE in vivo warrant further investigation. In conclusion, magnetic antibody-linked nanomatchmakers enable molecular targeting, physical enrichment and noninvasive imaging all in one easily synthesized particle. By varying the antibodies and/or adding a drug payload onto the iron core, the strategy is broadly generalizable. Moreover, translatability to patients should be straightforward, given that both the iron nanocore and the recombinant human antibodies are widely utilized clinically. Preparation and characterization of MagBICE MagBICE 1 was generated by conjugating rabbit anti-CD45 (Abcam) and mouse anti-MLC (Abcam) antibodies. MagBICE 2 was generated by conjugating anti-CD45 and goat anti-CD34 (LifeSpan Biosciences) antibodies to FH particles, using an EDAC-based PolyLink Coupling Linking Kit (Bangs Laboratories). Briefly, 50 μl of FH particles, 100 μg of anti-CD45 antibodies (or anti-CD34 antibodies), 100 μg of anti-MLC antibodies and 40 μl of EDAC were mixed in Protein Link Buffer and incubated at room temperature for 4 h with gentle rocking. After that, the whole contents were centrifuged at 13,000 r.p.m. for 10 min. The supernatants were removed and the resultant MagBICE particles were washed twice with Protein Wash/Storage Buffer and stored at 4 °C in the same buffer. Cryo-TEM was performed to visualize MagBICE [25] . Conjugated antibodies were negatively stained with uranyl acetate and iron oxide cores in the complex were unstained. To prepare grids, 3 μl aliquots of sample were placed on Quantifoil 2/1 Holey Carbon Film grids, blotted with filter paper and rapidly plunged into liquid ethane. Images were recorded in an FEI TF20 cryo-electron microscope operated at 200 kV. To confirm the presence of primary antibodies, MagBICE was incubated with goat-anti-mouse (Texas-Red, 2 mg ml −1 , 1:400 dilution; Abcam) and goat-anti-rabbit (FITC, 2 mg ml −1 , 1:400 dilution; Abcam) secondary antibodies, spun down and observed with a Nikon EclipseTE2000-U epi-fluorescence microscope. Conjugation efficiency was further assessed by SDS–PAGE and absorbance at 280 nm (A280) protein concentration measurement with a NanoDrop ND-100 Spectrophotometer (Thermo Scientific). Hydrodynamic size and zeta potential were measured with a Zetasizer Nano ZS90 (Malvern Instruments). In vitro cell binding and engaging studies Rat BMCs were derived from Wistar-Kyoto rats by femur and tibia bone flush and gradient centrifugation [26] . Rat NRCMs were derived and cultured as previously described [27] . Briefly, NRCMs were isolated from 1- to 2-day-old neonatal rat pups and cultured as a monolayer. The culture media was based on M199 (Life Technologies) with the following components: 10 mM HEPES, 0.1 mM non-essential amino acids, 3.5 mg ml −1 glucose, 2 mM L -glutamine, 4 μg ml −1 vitamin B12, 100 U ml −1 penicillin and heat-inactivated FBS at 10% (first 2 days of culture) or 2% (after 2 days of culture) final concentration. Rat BMCs were incubated with MagBICE 1 or unconjugated FH for 15 min at 37 °C. After wash, the cells were further incubated with goat-anti rabbit FITC antibodies for 15 min at 37 °C. Binding efficiency was checked by a Leica TCS SP5 X confocal microscopic system and a Cyan flow cytometry (Beckman-Coulter) with Summit Software. Prussian blue staining [13] was performed to visualize iron on BMCs and an antibody stripping protocol [28] was employed to rule out endocytosis of iron by BMCs. To create injured cardiomyocytes in vitro , NRCMs were briefly permeabilized for 5 min at 4 °C with BD Cytofix/Cytoperm fixation and permeabilization solution (BD). After wash, the injured cells were incubated with MagBICE 1 or unconjugated FH for 1 h at 37 °C and further incubated with fluorescent secondary antibodies for 1 h at 37 °C. The cells were then observed under a Leica TCS SP5 X confocal microscopic system (Leica). To demonstrate conjoining, rat BMCs were labelled with a fluorescent dye (DiD; Invitrogen) and co-cultured with injured NRCMs for 1 h, in the presence of MagBICE 1 or FH. After extensive wash, the BMCs attaching to the injured NRCMs were quantified. In vitro cytotoxicity studies For cardiomyocyte viability assay, rat NRCMS were incubated with 60 μg iron per ml MagBICE 1 or unconjugated FH for 24 h at 37 °C. The cell cultures were then washed and stained with a LIVE/DEAD Viability/Cytotoxicity Kit (Invitrogen) [29] , which quickly discriminates live from dead cells by simultaneously staining with green-fluorescent calcein-AM (live) and red-fluorescent ethidium homodimer-1 (EthD; dead). Rat BMC proliferation in the presence of MagBICE 1 or FH was assessed by a Cell Counting Kit-8 (CCK-8; Dojindo Molecular Technologies) [30] . BMC migration in the presence of MagBICE 1 or FH was evaluated with a transwell cell migration assay plate (BD Biosciences) [31] . In vivo binding studies All animal procedures were in accordance with the Cedars-Sinai Institutional Animal Care and Use Committee. MI was created in 8- to 12-week female Wistar-Kyoto rats by 3 h ischemia and 20 min reperfusion [30] . Saline (400 μl PBS), unconjugated FH (10 mg iron per kg body weight in 400 μl PBS) or MagBICE (10 mg iron per kg body weight in 400 μl PBS) was intravenously infused through tail veins. Twenty-four hours after infusion, MRI of the heart was accomplished by a gradient echo sequence to produce a T 2 * weighting with a Bruker Biospec 9.4T small animal MRI system (Bruker). A 60-mm diameter linear transmit/receive coil (Bruker, T10325V3) was utilized for excitation and a 4-channel array coil (Bruker, T10324V3) designed for rat heart imaging was used for improved signal-to-noise data acquisition. The pulse sequence details are the repetition time (TR): 5.1 ms; the echo time (TE): 2.4 ms; the flip angle (FA): 8.0°. Retrospective gating was accomplished with Bruker IntraGate software (Bruker) to produce ten cine images for each slice. In addition, one coronal cine image was acquired, which dissected the heart to verify the presence of iron particles. Iron signal intensity was quantified from the transverse images with NIH ImageJ software and normalized to adjacent tissues. After the imaging session, animals were euthanized and 8-μm-thick heart cryo-sections were prepared using a microtome. To visualize the retention of MagBICE 1 particles in the heart and its co-localization with cardiomycytes, the sections were fixed with 4% paraformaldehyde, permeablized/blocked with Protein Block Solution (DAKO) containing 1% saponin (Sigma) and stained with FITC-conjugated secondary antibodies (to detect the primary antibodies on MagBICE 1 ) and alpha-sarcomeric actin (Abcam; detected by Texas-Red-conjugated secondary antibodies). Images were taken by a Leica TCS SP5 X confocal microscopy system. The targeting efficiency of MagBICE 1 was quantified by the FITC signal intensity normalized to the Texas-Red signal intensity of the same field, using the Leica LAS AF Software. The presence of iron was further confirmed by tissue Prussian blue staining [30] . Slides were also stained with FITC-conjugated anti-CD45 (Abcam) or Cy5-conjugated anti-CD68 antibodies (Abcam) to evaluate whether MagBICE 1 targets endogenous cells and/or exacerbated inflammation in the post-MI heart. To examine whether endogenous stem cells are captured by infused MagBICE 2 (CD34-Fe-MLC), PBMCs were isolated from unconjugated FH- and MagBICE 2 -infused animals using Ficoll density gradient centrifugation 24 h after treatment. The PBMCs were magnetically sorted for iron-bound (MagBICE or FH) cells. The positive populations were analysed for CD34 expression by flow cytometry. Iron overload studies Day 3 after MagBICE 1 or FH infusions, subpopulations of animals were used for iron overload studies. Serum transferrin and ferritin levels were measure by commercially available ELISA kits (Rat Transferrin and Rat Ferritin, Immunology Consultants Laboratory Inc., cat# E-25TX and E-25F) [28] . Liver histology was performed to assess excessive amount of free iron deposition by Prussian blue staining [30] . Therapeutic efficacy study In a similar rat ischemia/reperfusion injury model, MagBICE 1 or unconjugated FH were intravenously infused into 6- to 8-week-old female Wistar-Kyoto rats. In addition, 2 million DiI-labelled BMCs (from male rats) were intravenously infused 20 min after nanoparticle infusion. A saline-only group was included as control. Twenty-four hours after nanoparticle/cell infusion, subpopulations of animals from each group were killed. Hearts/lungs/livers were excised, washed with saline and subjected to ex vivo fluorescent imaging using an IVIS 200 (Xenogen) system to measure the DiI fluorescence. Fluorescent signal (total flux (p s −1 )) was quantified as described [13] . BMCs were quantified in heart cryo-sections by counting the DiI-positive cells. Cell nuclei were counter-stained with 4′,6-diamidino-2-phenylindole and MagBICE 1 was visualized by FITC-conjugated anti-rabbit secondary antibodies. Rats underwent echocardiography 24 h (baseline) and 4 weeks post MI using Vevo 770 Imaging System (VisualSonics) [32] . Hearts were imaged two-dimensionally in long-axis views at the level of the greatest LV diameter. LVEF was measured with VisualSonics V1.3.8 software from views taken through the infarcted area. After the echocardiography session at 4 weeks, all animals were killed for histology studies. Masson’s trichrome staining was performed as per manufacturer’s instructions (HT15 Trichrome Staining (Masson) Kit; Sigma). Images were acquired with a PathScan Enabler IV slide scanner (Advanced Imaging Concepts). From the Masson’s trichrome-stained images, infarct wall thickness was measured with NIH ImageJ software [13] and volumetric analyses of viable mass, scar mass and scar size were performed [33] . To quantify the level of angiogenesis in the infarct zone, slides were stained with anti-smooth muscle actin and the smooth muscle actin-positive arteriolar structures were counted. Magnetic enrichment experiment MagBICE 2 (10 mg iron per kg body weight in 400 μl PBS) was intravenously infused through the tail veins of healthy Wistat-Kyoto rats, with a 1.3-T circular neodymium magnet placed above the left thoracic region during infusion and continuously for 10 min after infusion [30] . After, the animal was imaged with a Bruker Biospec 9.4T small animal MRI system to track the distribution of infused MagBICE particles. Statistical analysis Results are presented as mean±s.d. unless specified otherwise. Comparisons between any two groups were performed using two-tailed unpaired Student’s t -test. Comparisons among more than two groups were performed using one-way ANOVA followed by post-hoc Bonferroni test. Differences were considered statistically significant when P <0.05. How to cite this article: Cheng, K. et al . Magnetic antibody-linked nanomatchmakers for therapeutic cell targeting. Nat. Commun. 5:4880 doi: 10.1038/ncomms5880 (2014).